Bioinspired hollow semiconductor nanospheres as photosynthetic nanoparticles Natural photosynthesis occurs in the thylakoid membrane where functional proteins and electron carriers are precisely arranged to efficiently convert sunlight into a chemical potential between the two membrane sides, via charge separation and electron transport chains, for use in oxygen generation and CO 2 fixation. These light-harvesting complexes and cofactors have been actively mimicked using dyes, semiconductors and catalytic nanoparticles. However, the photosynthetic scaffold that optimizes both the capture and distribution of light and separates both the oxidative and reductive species has been mimicked much less often, especially using polymer substances. Here we report the synthesis of hollow nanospheres sized in the optical range and made of a robust semiconductor, melon or carbon-nitride polymer. These hollow nanospheres are shown to function as both light-harvesting antennae and nanostructured scaffolds that improve photoredox catalysis, which was determined to have a 7.5% apparent quantum yield via a hydrogen-generation assay. Hollow nanostructured materials mimicking vesicles and cells have attracted attention for many years as their unique structural, physical and chemical properties have potential applications in drug delivery, catalysis, gas storage, lithium batteries and nanodevices [1] , [2] , [3] . Polymerized hollow nanospheres with controlled surface functionalities are particularly interesting because they can act as scaffolds that coassemble various functional motifs into complex nanostructures while maintaining an 'interior' and 'exterior' with a 'membrane' separating the two. An analogy in nature is the photosynthetic thylakoid membrane where both the water-oxidation centre (photosystem II) and carbon dioxide-reduction centre (photosystem I) are cooperatively organized for highly efficient energy conversion and transfer through photon conversions in the nanosized structure [4] . It is also known that photooxidation and photoreduction are locally incompatible and must be strictly separated in nanospace. Their placement on two sides of a membrane enables a local proton gradient to develop, which drives adenosine triphosphate synthesis via the photoredox reactions. This process has stimulated intense research to understand and even mimic such biological energy-transfer processes in man-made, three-dimensional nanoarchitectures; however, the high complexity of biology still challenges material designers. When expanding upon nature via biomimetics [5] , the choice of materials is not confined by biology. For hollow nanospheres inspired by thylakoids, it is particularly interesting for the shell to be constructed from organic semiconductors, such as conjugated polymers, developed for plastic (opto)electrics [6] , [7] . These materials would allow for the direct generation of the reactive electrons and holes on the shell with sufficient energy for redox chemistry without relying on chromophoric molecules that need to be grafted onto the surface via complicated chemical designs and syntheses. A range of inorganic hollow structures have been synthesized via templated methods employing polymer latex [8] , [9] , silica [10] , [11] , acoustic bubbles [12] and emulsion/microemulsion [13] as the templates, and some of these spherical and hollow semiconductor structures have been used for the photocatalytic splitting of water [14] , [15] , [16] . Nevertheless, the templated synthesis of robust conjugated polymer hollow nanospheres with a shell thickness of <100 nm is rarely covered. The difficulty in fabricating polymeric hollow nanospheres is partly due to the ease of deforming their hollow nanostructures after template and solvent removal, even when the polymer is highly cross-linked [17] . However, once these conjugated vesicles have been successfully fabricated, they can act as a 'plugboard' for designing complex nanoarchitectures, with large surface areas for both their exterior and interior that increase the amount of light absorbed by the photonic effects and promote surface-dependent reactions by efficiently shuttling both the electronic and chemical species. Such materials show good promise for heterogeneous (photo)chemical applications. In principal, the optoelectric properties of an organic semiconductor are related to the binding energy ( E b ) of its Frenkel-type excitons, which decreases from its quasi-one-dimensional value to the two- and three-dimensional values [18] . It is therefore highly desirable to construct conjugated polymers that are planar, two-dimensional, rather than a linear-backbone, one-dimensional, to facilitate exciton splitting, which is regarded as the key step for improving the overall performance of polymer photovoltaic devices [19] . Here we report a simple hard-templating approach to synthesizing polymeric hollow nanospheres of graphitic carbon nitride (g-C 3 N 4 ) constructed from N-bridged tri- s -triazine repeating units that form two-dimensional conjugated planes packed together via Van der Waals interactions [20] , [21] , [22] , [23] . The tri- s -triazine ring structure makes the polymer practically inert to chemical attacks (for example, acid, base, oxygen and organic solvents) and provides an appealing electronic structure as well as surface basicity [24] . These properties have already enabled its use for applications in the energy, catalysis and environmental fields, such as water splitting [25] , [26] , [27] , oxygen-reduction reactions [28] , [29] , selective hydrocarbon oxidation [30] , [31] , carbon dioxide activation [32] and pollutant control [33] . An improvement to these material functions once this earth-abundant organic semiconductor has been fabricated as a hollow nanostructure with controlled dimensions and surface functionalities can be predicted [34] , [35] . Herein, we use a nanostructured silica template to fabricate highly stable, hollow carbon nitride nanosphere (HCNS) with controlled shell thicknesses as a light-harvesting platform for catalysing hydrogen evolution under visible light irradiation and achieved a 7.5% overall apparent quantum yield (AQY). The fabrication of nanostructured silica templates and HCNS Homodisperse silica particles were synthesized as a sacrificial core material according to the Stöber method using tetraethoxysilane (TEOS) as the precursor. After the SiO 2 core had formed, another batch of TEOS was added with n -octadecyltrimethoxysilane (C 18 TMOS) as a porogen and calcined at 550 °C to generate a thin mesoporous silica shell. The thickness of the mesoporous silica shell can be controlled by adjusting the amount of TEOS and C 18 TMOS added to the SiO 2 cores in an ethanol, water and aqueous ammonia solution. These monodisperse silica nanoparticles were then used as a template to make HCNS and functionalised HCNS as illustrated in Fig. 1 . Briefly, cyanamide (CY) was loaded into the pores of the mesoporous silica shell to obtain CY/silica hybrids that were subsequently converted to g-C 3 N 4 /silica nanocomposites via the thermal-induced self-condensation of CY at 550 °C before removing the silica template with NH 4 HF 2 (for more details, see the Supplementary Information ). The obtained HCNSs were denoted as HCNS- X , where X is an arbitrary sample number that represent the different shell thicknesses. The HCNS- X samples were characterized with respect to their local order, chemical structure, semiconductor properties and performance for photocatalytic hydrogen evolution after creating a surface metal/semiconductor heterojunction via in situ light-induced catalytic deposition. 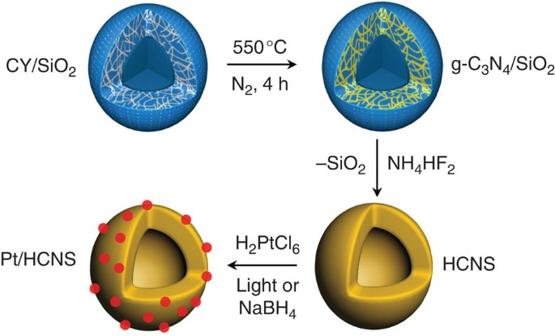Figure 1: Synthetic strategy. An illustration of the HCNS and metal/HCNS composite syntheses. Figure 1: Synthetic strategy. An illustration of the HCNS and metal/HCNS composite syntheses. Full size image Characterization of the crystal and chemical structures X-ray diffraction (XRD) patterns and both Fourier transform infrared (FTIR) spectroscopy and solid-state 13 C cross-polarisation nuclear magnetic resonance (CP-NMR) spectra were used to determine the chemical structure and local order of representative HCNS samples with a shell thickness of ~56 nm. As shown in Fig. 2a , the XRD peak at 27.6° is attributed to the (002) reflection of a graphitic-like aromatic structure with a d -value of 0.323 nm, whereas the peak at 13.1° corresponds to the in-plane repeating motifs of the continuous heptazine network [20] , [21] , [22] , [23] , [24] . Higher quality condensations can be indirectly detected by improved packing in the (002) direction of the XRD patterns ( Fig. 2a ). The (002) reflection peak for the HCNS sample shifted from 27.3 (bulk g-C 3 N 4 ) to 27.6°, that is, the average inter-plane distance of the HCNS compressed from 0.326 (bulk g-C 3 N 4 ) to 0.323 nm. The band at 810 cm −1 in the FTIR spectrum shown in Fig. 2b belongs to the s -triazine ring modes, and the bands at 1,200–1,600 cm −1 are characteristic of aromatic CN heterocycles [20] , [21] , [22] , [23] , [24] . The solid-state 13 C CP-NMR spectra ( Fig. 2c ) further confirms the presence of heptazine tectons in the g-C 3 N 4 solids, and the signals at approximately 155.6 and 164.3 ppm related to the formation of a poly(tri- s -triazine) structure characteristic of melem, melon and the final carbon nitride [21] , [36] , [37] . The presence of sharper lines in the NMR spectrum of the HCNS sample than the bulk g-C 3 N 4 could be due to a reduced inhomogeneous broadening of the hollow sphere samples, which would indicate an improved condensation and local organization in the thin shell structure. 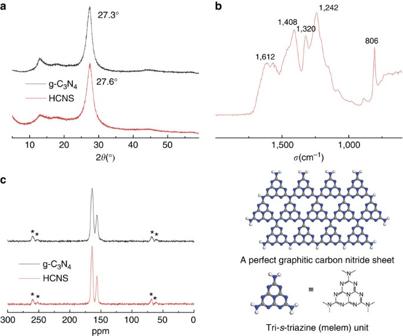Figure 2: Structure characterizations of a representative hollow carbon nitride sphere. (a) XRD pattern. (b) FTIR profiles. (c) Solid-state13C NMR spectrum of a molecular g-C3N4structure based on poly(tri-s-triazine) motifs. *Indicates the spinning side bands in the13C spectra. Figure 2: Structure characterizations of a representative hollow carbon nitride sphere. ( a ) XRD pattern. ( b ) FTIR profiles. ( c ) Solid-state 13 C NMR spectrum of a molecular g-C 3 N 4 structure based on poly(tri-s-triazine) motifs. *Indicates the spinning side bands in the 13 C spectra. Full size image Note that all XRD, FTIR and NMR spectra of the HCNS samples resemble the reference g-C 3 N 4 sample, which suggests that the g-C 3 N 4 -based nanostructures were successfully fabricated via the hierarchical templating method. Morphological investigations Both scanning emission microscope and transmission electron microscope (TEM) images ( Supple-mentary Fig. S1a ) of the silica templates indicated uniform nanostructured silica particles with a ~220-nm condensed core and a controlled porous shell 20–100 nm thick based on the amount of TEOS and C 18 TMOS added. The particle size was chosen to be similar to the optical bandgap of the carbon nitride semiconductor, which is <~430 nm. Having a wavelength-scale particle size and shell thickness maximize the light harvesting via inner reflections and photonic effects within the carbon nitride nanostructures [38] . Removing both the dense silica core and porous silica shell yields a hollow carbon nitride vesicle ( Fig. 3a–f ) that inherited most of its geometrical features from the parent SiO 2 nanostructures. The thickness of the HCNS shell is strongly related to the thickness of the mesoporous SiO 2 layer over the dense SiO 2 cores ( Supplementary Fig. S1b ). It should be noted that we found few mesopores in the carbon nitride shell, presumably because of the collapse of the carbon nitride polymers upon removing the mesoporous silica shell. Indeed, the irreversible deformation/collapse of the central cavity into a bowl-like morphology also occurred when the polymeric shell thickness approached 56 nm, as the capillary stress became too high to preserve the spherical shape of such a soft material [17] , [39] , [40] . Hollow structures with a shell thickness of ~<30 nm are found to almost completely collapse after template removal ( Supplementary Figs S2e and f ). Intact hollow nanospheres with a shell thickness of ~60 nm that are monodisperse in both their outer and inner diameter could be reproducibly obtained even after being dried at 400 °C in air for 2 h ( Fig. 3h ; Supplementary Fig. S3 ). This finding reveals the robust and thermally stable nature of the HCNS sample. 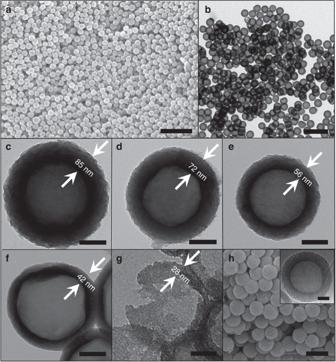Figure 3: Surface morphology of hollow carbon nitride spheres. (a) The large-area scanning emission microscope (SEM) of HCNS-3; the scale bar equals 2 μm. (b) The large-area TEM of HCNS-3; the scale bar equals 1 μm. (c–g) TEM images of HCNS-1 to -5 with different shell thicknesses; the scale bar equals 100 nm. (h) SEM image of HCNS-3 after heating at 400 °C in air for 2 h, with an inset showing the corresponding individual hollow sphere in TEM; scale bar equals 0.5 μm, and the inset scale bar equals 100 nm. Figure 3: Surface morphology of hollow carbon nitride spheres. ( a ) The large-area scanning emission microscope (SEM) of HCNS-3; the scale bar equals 2 μm. ( b ) The large-area TEM of HCNS-3; the scale bar equals 1 μm. ( c – g ) TEM images of HCNS-1 to -5 with different shell thicknesses; the scale bar equals 100 nm. ( h ) SEM image of HCNS-3 after heating at 400 °C in air for 2 h, with an inset showing the corresponding individual hollow sphere in TEM; scale bar equals 0.5 μm, and the inset scale bar equals 100 nm. Full size image Evolution of the semiconductor band structure It is known that the semiconductor structure of g-C 3 N 4 originates from the formation of s -triazine units into an extended π-conjugated system, which depends on their extent of polymerization [24] . The evolution of the band structure for CN precursors condensed at different temperatures was monitored using their electron paramagnetic resonance (EPR) spectra ( Fig. 4a ), which yields a g value of 2.0034 for the delocalized electrons in the conduction band of a carbon nitride semiconductor [41] . There was no EPR signal for melamine and melem, whereas a peak began to evolve at 450 °C, which indicates the beginning of the polymerization (development of the band structure). Well-resolved EPR signals were observed at >530 °C; therefore, an electronic band structure in the HCNSs was established at 550 °C. The spin intensity of the HCNS samples increased upon light excitation, indicating that the charge radicals were generated on the organic semiconductor. 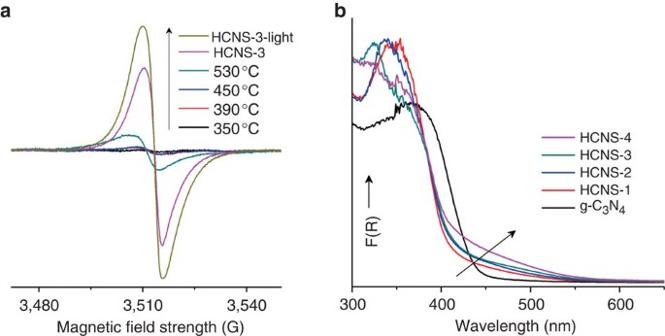Figure 4: Electronic structure and optical absorption of hollow carbon nitride spheres. (a) EPR spectrum of carbon nitride solids condensed at different temperatures. (b) Optical absorption of the g-C3N4and HCNS samples. Figure 4: Electronic structure and optical absorption of hollow carbon nitride spheres. ( a ) EPR spectrum of carbon nitride solids condensed at different temperatures. ( b ) Optical absorption of the g-C 3 N 4 and HCNS samples. Full size image Optical absorption properties The formation of an electronic band structure was further indicated by the semiconductor-like optical absorption ( Fig. 4b ). The abrupt onset of absorption at ~430 nm is due to the electronic transition from the valance band to the conduction band in the carbon nitride semiconductor upon excitation with light. The enhanced light absorption in the range of 440–550 nm for the HCNS samples over the bulk g-C 3 N 4 is believed to reflect the ability of the hollow nanospheres to have multiple reflections within the structure, which increases the effective path length for light absorption. However, this enhanced light harvesting in the visible light range may also be due to an increasing number of defects in the material upon decreasing the shell thickness into the nano range [25] . It was noted that the optical absorption of the HCNS samples shifted to the blue, which might also be due to a quantum size effect [25] , [42] . These findings translate to a higher redox power for the photogenerated e/h pairs for the HCNS samples relative to the reference g-C 3 N 4 . Photocatalytic properties A light-induced hydrogen-evolution assay was conducted on the HCNS samples using 3 wt% Pt as the cocatalyst. All of the HCNS samples exhibited enhanced photocatalytic activity over bulk Pt/g-C 3 N 4 for hydrogen evolution ( Supplementary Fig. S4 ). The initial hydrogen-evolution rate (HER) for Pt/HCNS-1 was 224 μmol h −1 , which is a factor of 25 higher than that of the bulk phase (9 μmol h −1 ). The AQY of Pt/HCNS-1 (with a performance of 224 μmol H 2 h −1 ) is estimated to be 7.5%, which is comparable to and outperforms the various benchmark inorganic photocatalysts (like TiO 2 and N-doped TiO 2 ) under UV and visible light irradiation, respectively ( Supplementary Table S1 ) [43] , [44] , [45] . The HER of the Pt/HCNS-1-to-4 samples gradually and unexpectedly decreases with decreasing shell thickness, though the surface area of the samples increases. The optimal size of a nanostructure in organic electronics is related to the mean free migration path of any photo-induced charges, which is generally expected to be in 10–30 nm range. However, the defect number can also increase with decreasing shell thickness, which potentially makes the effectiveness a balance between two counteracting effects. Note that the HER of Pt/HCNS-5 abruptly decreased to 23 μmol H 2 h −1 when the nanostructure was seriously deformed (as confirmed by the rapid decrease of the surface area to 37 m 2 g −1 in Table 1 ), which again indicates the advantage of an intact hollow nanostructure with a proper shell thickness for heterogeneous photochemical applications. The stability of the Pt/HCNS sample under light and in contact with water was examined by repeatedly conducting the hydrogen-evolution experiments. As shown in Fig. 5 , the material still maintained most of its intrinsic photocatalytic activity after seven cycles. The TEM image of the used HCNS depicted an apparently unaltered hollow nanosphere ( Fig. 6 ) with the exception of some dark spots formed on the surface due to the in situ deposition of Pt nanoparticles as a cocatalyst and hydrogen-evolution site [9] . The FTIR spectrum after the reaction remained unchanged ( Supplementary Fig. S5 ). These results provide directly proof of the stability of the phase and both textural and surface structures of the HCNSs under the applied reaction conditions. Table 1 Physical and photochemical properties. 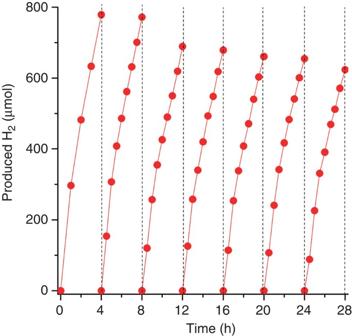Figure 5: Stability of HCNS during prolonged photocatalytic operation. The photocatalytic stability test of the 3 wt% Pt/HCNS-3 (50 mg) sample over seven repeated operations under visible light (λ>420 nm) in contact with water. The total H2gas production across the seven runs was 109 cm3, and the corresponding turnover number with respect to the polymer and Pt was 17.9 and 633, respectively, confirming the photocatalytic nature of the system. Full size table Figure 5: Stability of HCNS during prolonged photocatalytic operation. The photocatalytic stability test of the 3 wt% Pt/HCNS-3 (50 mg) sample over seven repeated operations under visible light ( λ >420 nm) in contact with water. The total H 2 gas production across the seven runs was 109 cm 3 , and the corresponding turnover number with respect to the polymer and Pt was 17.9 and 633, respectively, confirming the photocatalytic nature of the system. 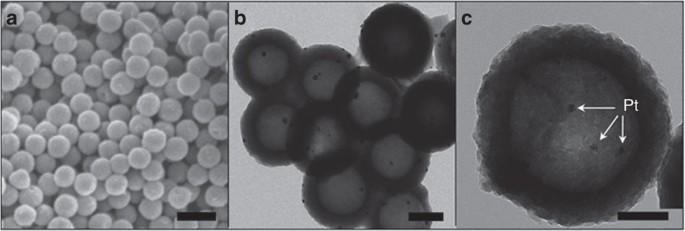Figure 6: Morphology of hollow carbon nitride spheres after the photochemical reaction. (a) SEM and (b,c) TEM images of HCNS-1 after the photocatalytic reaction under visible light irradiation. The scale bars ina,bandcare 500, 200 and 100 nm, respectively. Full size image Figure 6: Morphology of hollow carbon nitride spheres after the photochemical reaction. ( a ) SEM and ( b , c ) TEM images of HCNS-1 after the photocatalytic reaction under visible light irradiation. The scale bars in a , b and c are 500, 200 and 100 nm, respectively. Full size image In summary, hollow g-C 3 N 4 nanospheres have been successfully synthesized using silica nanoparticles as templates. Carefully controlling the shell thickness of the polymeric hollow nanospheres prevents the deformation of the soft hollow structure, even after sintering at 400 °C. The application of these mono-disperse hollow conjugated semiconductor vesicles has been demonstrated using a photocatalytic hydrogen-evolution assay, and their advantages from the inner optical reflection and improved structure condensation provide a remarkably increased photochemical activity, reaching an overall AQY of approximately 7.5%. Although the blue shift of the band gap, which was associated to either a quantum size effect or enhanced H-type interlayer packing, was unwanted, further chemical control, such as extending the pi system by anchoring aromatic motifs, are already available to expand the visible absorption, for example, through copolymerisation [46] , [47] . Hybrid nanoarchitectures based on finely tuned polymeric carbon nitride capsules provide a valuable platform for constructing highly organized photosynthetic systems for the efficient and sustained utilization of solar radiation after the controlled deposition of a cocatalyst onto the exterior and/or interior surfaces and the construction of a dyadic layer to promote exciton dissociation. Synthesis of the SiO 2 template A dense monodisperse silica core covered with a thin mesoporous silica shell was used as a template to synthesize the hollow carbon nitride spheres. In detail, 3.10 g of aqueous ammonia (32 wt%) were added to an ethanol solution containing 58.5 g of ethanol and 10 g of deionised water. After stirring for 30 min at 30 °C, 5.6 ml of TEOS was added to the above mixture with vigorous stirring and was left stationary for 1 h to yield uniform nonporous silica spheres (Stöber silica sol). A mixture of TEOS and C 18 TMOS was then added dropwise to the above solution with magnetic stirring to create a thin mesoporous silica shell around the dense silica core. The thickness of this mesoporous silica shell can be adjusted by adding different amounts of TEOS and C 18 TMOS (see Table 1 ). The mixed solution was then kept at ambient temperature for 3 h without stirring to promote the cohydrolysis and condensation of the TEOS and C 18 TMOS on the nonporous SiO 2 beads. The nanostructured silica was centrifuged, dried at 70 °C and calcined at 550 °C for 6 h in air. The as-prepared monodisperse SiO 2 templates were neutralized with a 1-M HCl solution and then dried at 80 °C overnight to obtain the final silica template. Synthesis of HCNS A solution of 2 g of the SiO 2 template and 10 g of CY was mixed for 3 h in a flask connected to a vacuum line before subjecting to sonication at 60 °C for 2 h. Afterwards, the mixture was stirred at 60 °C overnight. The resultant mixture was centrifuged and dried in air to obtain a white solid that was transferred to a crucible and heated to 550 °C under flowing N 2 for 4 h with a ramp rate of 4.4 °C min −1 . The obtained yellow g-C 3 N 4 /SiO 2 hybrids were treated with 4 M NH 4 HF 2 for 12 h to remove the silica template. The powders were then centrifuged and washed three times with distilled water and once with ethanol. The final yellow HCNS powders were obtained by drying at 80 °C in a vacuum oven overnight. Synthesis of the bulk g-C 3 N 4 The bulk g-C 3 N 4 was synthesized as a reference sample by placing 2 g of CY in a crucible and heating to 550 °C under flowing N 2 for 4 h with a ramp rate of 4.4 °C min −1 (the same thermal treatment conditions as for the HCNS synthesis). Characterization Powder XRD measurements were performed on a Bruker D8 Advance diffractometer using CuK-α1 radiation ( λ =1.5406 Å). The FTIR spectra were collected using a Varian 1000 FTIR spectrometer. The optical absorption measurements were collected using a Varian Cary 500 Scan UV-visible system. The TEM images were obtained using a Zeiss EM 912 TEM. The scanning emission microscope measurements were conducted using a Zeiss LEO 1550 Field Emission Scanning Electron Microscope. Nitrogen adsorption–desorption isotherms were collected at 77 K using a Micromeritics ASAP 2020 Analyser. EPR measurements were conducted on a Bruker A300 Spectrometer Model. The solid-state CP-NMR spectra were collected using a Bruker Advance III 500 Spectrometer. Performance analysis Photocatalytic H 2 production was measured in a Pyrex top-irradiation reaction vessel connected to a glass-closed gas-circulation system. For each reaction, a certain amount of the photocatalyst powder was dispersed in 100 ml of an aqueous 10% triethanolamine scavenger solution by volume. H 2 PtCl 6 dissolved in the reactant solution was used to photodeposit 3 wt% of Pt onto the catalysts. The reactant solution was evacuated several times to completely remove air before irradiation under a LX300F 300 W Xe-lamp (Shenzhen ShengKang Technology) and water-cooling filter. The wavelength of the incident light was controlled using an appropriate long pass cut-off filter. The reaction solution was maintained at room temperature using a flow of cooling water during the reaction. The evolved gases were analysed using a gas chromatograph (Shimadzu GC-8A) equipped with a thermal conductive detector. The AQY for the H 2 evolution was measured using a similar experimental setup, only with a band pass filter ( λ =420.5 nm with the photon flux of 49.4 mW cm −2 ) and was estimated as follows: where R and I represent the rates of H 2 evolution and the number of incident photons, respectively. The total number of incident photons was measured using a calibrated silicon photodiode. How to cite this article: Sun, J. et al. Bioinspired hollow semiconductor nanospheres as photosynthetic nanoparticles. Nat. Commun. 3:1139 doi: 10.1038/ncomms2152 (2012).